An efficient molybdenum disulfide/cobalt diselenide hybrid catalyst for electrochemical hydrogen generation The electroreduction of water for sustainable hydrogen production is a critical component of several developing clean-energy technologies, such as water splitting and fuel cells. However, finding a cheap and efficient alternative catalyst to replace currently used platinum-based catalysts is still a prerequisite for the commercialization of these technologies. Here we report a robust and highly active catalyst for hydrogen evolution reaction that is constructed by in situ growth of molybdenum disulfide on the surface of cobalt diselenide. In acidic media, the molybdenum disulfide/cobalt diselenide catalyst exhibits fast hydrogen evolution kinetics with onset potential of −11 mV and Tafel slope of 36 mV per decade, which is the best among the non-noble metal hydrogen evolution catalysts and even approaches to the commercial platinum/carbon catalyst. The high hydrogen evolution activity of molybdenum disulfide/cobalt diselenide hybrid is likely due to the electrocatalytic synergistic effects between hydrogen evolution-active molybdenum disulfide and cobalt diselenide materials and the much increased catalytic sites. Owing to their diffuse nature, electricity from renewable but intermittent energy (for example, solar and wind) must be stored durably for off-grid applications. Electrochemical water splitting to produce hydrogen (H 2 ) offers a promising and sustainable solution for this purpose by converting such electricity energy into stable chemical bonds [1] , [2] . Appropriate electrocatalysts, such as platinum (Pt) and its alloys, play a vital role in the H 2 evolution reaction (HER) because they can catalyse the conversion from a pair of protons and electrons to H 2 at high reaction rates and low overpotentials ( η ) [1] , [2] , [3] . However, the prohibitive cost and scarcity of Pt pose tremendous limitations to widespread use. Therefore, finding robust and efficient alternative catalysts that are geologically abundant is crucial to the future of ‘hydrogen economy’. Molybdenum disulfide (MoS 2 ), a widely used industrial catalyst for hydrodesulfurization [4] , has recently demonstrated promise as effective HER catalyst based on both computational and experimental studies [5] , [6] . The HER activity was discovered to arise from the exposed (10–10) planes on edges of MoS 2 , whereas the (0001) basal planes are catalytically inactive [5] , [6] , [7] . This understanding has led to great efforts to develop highly nanostructured MoS 2 -based HER catalysts to maximize the number of edge sites, including crystalline [8] , [9] , [10] , [11] , [12] and amorphous materials [13] , [14] , [15] , MoS 2 -based hybrid materials [16] , [17] , [18] , [19] and molecular mimics [7] . Despite significant success, the design and fabrication of MoS 2 -based HER electrocatalysts with satisfactory activity and stability remain a big challenge. In recent years, we have been making efforts to explore efficient electrocatalysts by using Earth-abundant 3 d metal (Co, Ni and so on) chalcogenides [20] , [21] , [22] , [23] , [24] , [25] , [26] , [27] . New NiSe nanofibres [24] and lamellar mesostructured CoSe 2 /DETA (DETA, diethylenetriamine) nanobelts [25] were found to show decent HER activity in acidic electrolyte. Kong et al. [28] also observed good HER activities from various polycrystalline transition metal dichalcogenide (ME 2 , M=Fe, Co, Ni; E=S, Se) films, especially from the CoSe 2 . Recently, we found that the HER activity of CoSe 2 nanobelts can be improved greatly after anchoring Ni/NiO nanoparticles onto their surfaces [25] . The synergetic chemical coupling effects between CoSe 2 and grafted Ni/NiO were believed to contribute to the enhancement. Similar promoted performances have also been observed on MoS 2 /graphene [16] , [17] , MoO 3 /MoS 2 (ref. 18 ) and MoS 2 /Au (ref. 19 ) composite catalysts for H 2 production. These works point to the possibility to access new and efficient HER catalysts by combining the promising CoSe 2 and MoS 2 . We report here that a HER electrocatalyst based on quasi-amorphous MoS 2 -coated CoSe 2 (denoted as MoS 2 /CoSe 2 ) hybrid is highly active and stable in acidic electrolyte. Notably, without any noble metals, the MoS 2 /CoSe 2 hybrid catalyst shows an onset potential close to commercial Pt catalyst (Johnson-Matthey, 20 wt% Pt/XC-72) and a small Tafel slope of ~36 mV per decade as well as no current loss after long-term chronoamperometry measurement, performing the best among the noble-metal-free HER electrocatalysts. These results suggest a strategy for designing non-noble metal catalysts with enhanced HER performance that is comparable to the state-of-the-art Pt-based catalysts. MoS 2 /CoSe 2 hybrid catalyst The MoS 2 /CoSe 2 hybrid was prepared directly in a closed N , N -dimethylformamide (DMF)/hydrazine solvothermal system, where (NH 4 ) 2 MoS 4 was used as a precursor for growing MoS 2 around the freshly made CoSe 2 /DETA nanobelt substrates ( Fig. 1a ; Supplementary Fig. 1 ; see Methods for details of the synthesis). The MoS 2 -coated CoSe 2 hybrid was shown by means of scanning electron microscopy and transmission electron microscopy (TEM; Fig. 2a–c ), which revealed the compact graphene-like MoS 2 nanosheets grown on the surface of CoSe 2 with a partially free-standing branch-like feature ( Supplementary Fig. 2 ). Substantial amino groups on the CoSe 2 /DETA surface ( Supplementary Fig. 3 ) serve as nucleation sites for coupling Mo precursor and subsequently reduced to MoS 2 on CoSe 2 (refs 21 , 23 ). A control experiment performed under identical synthesis conditions, but without CoSe 2 nanobelts, produced three-dimensional (3D) aggregates of MoS 2 sheets ( Fig. 1b ; Supplementary Fig. 4 ), suggesting that CoSe 2 could be a useful support for mediating the growth of loaded materials and constructing novel functional hybrids. 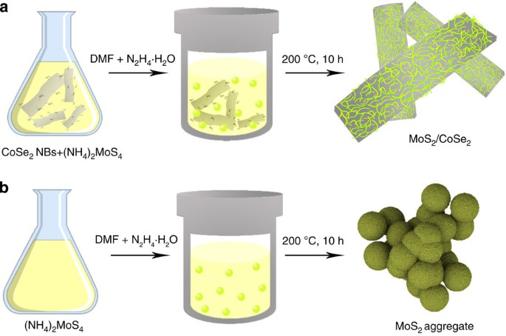Figure 1: Schematic illustration of the preparation of MoS2/CoSe2hybrid. (a) Solvothermal synthesis with CoSe2/DETA nanobelts as substrates for preparation of MoS2/CoSe2hybrid. (b) Solvothermal synthesis without CoSe2/DETA nanobelts leads to free MoS2nanosheet aggregates. Figure 1: Schematic illustration of the preparation of MoS 2 /CoSe 2 hybrid. ( a ) Solvothermal synthesis with CoSe 2 /DETA nanobelts as substrates for preparation of MoS 2 /CoSe 2 hybrid. ( b ) Solvothermal synthesis without CoSe 2 /DETA nanobelts leads to free MoS 2 nanosheet aggregates. 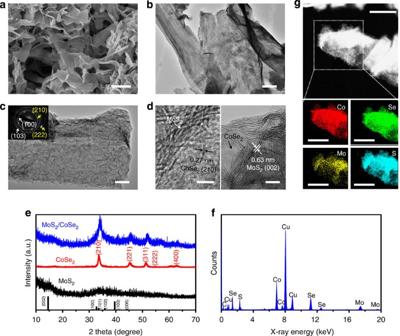Figure 2: Characterization of the MoS2/CoSe2hybrid. (a) Scanning electron microscopy image of MoS2/CoSe2hybrid. Scale bar, 800 nm. (b,c) TEM images with different magnifications of MoS2/CoSe2hybrid. Scale bars, 200 and 50 nm, respectively. The inset incshows corresponding SAED pattern. (d) HRTEM images of MoS2/CoSe2hybrid showing distinguishable microstructures of MoS2and CoSe2. Scale bars, 5 nm. (e,f) XRD patterns and EDX spectrum of the MoS2/CoSe2hybrid, respectively. (g) STEM-EDX elemental mapping of MoS2/CoSe2hybrid showing clearly the homogeneous distribution of Co (red), Se (green), Mo (yellow) and S (azure). Scale bars, 200 nm. Full size image Figure 2: Characterization of the MoS 2 /CoSe 2 hybrid. ( a ) Scanning electron microscopy image of MoS 2 /CoSe 2 hybrid. Scale bar, 800 nm. ( b , c ) TEM images with different magnifications of MoS 2 /CoSe 2 hybrid. Scale bars, 200 and 50 nm, respectively. The inset in c shows corresponding SAED pattern. ( d ) HRTEM images of MoS 2 /CoSe 2 hybrid showing distinguishable microstructures of MoS 2 and CoSe 2 . Scale bars, 5 nm. ( e , f ) XRD patterns and EDX spectrum of the MoS 2 /CoSe 2 hybrid, respectively. ( g ) STEM-EDX elemental mapping of MoS 2 /CoSe 2 hybrid showing clearly the homogeneous distribution of Co (red), Se (green), Mo (yellow) and S (azure). Scale bars, 200 nm. Full size image Figure 2d presents high-resolution TEM (HRTEM) images of the MoS 2 /CoSe 2 hybrid. Layered MoS 2 (often less than five layers) nanosheets, with an interlayer separation of 0.63 nm, were grown intimately on the CoSe 2 substrate. High-crystalline CoSe 2 substrate with d spacing of 0.27 nm can be seen frequently through the interspace of grafted MoS 2 (see Supplementary Fig. 5 for additional images). This non-fully covered structure may take advantage of merits from both MoS 2 and CoSe 2 for catalysing H 2 evolution. Selected area electron diffraction (SAED) pattern (inset in Fig. 2c ; Supplementary Fig. 6 ) revealed clear diffraction spots (marked by yellow arrows) from single-crystalline CoSe 2 support (JCPDS 9-0234) and also faint diffraction rings from grafted MoS 2 (JCPDS 77-1716). These barely recognizable diffraction rings indicate the quasi-amorphous structure of MoS 2 , consistent with the X-ray diffraction (XRD) data of MoS 2 /CoSe 2 with broadening diffraction peaks ( Fig. 2e ). Inasmuch as amorphous MoS 2 has recently been demonstrated to be effective HER catalysts [13] , [14] , [15] for its abundant defects and resultant more active edge sites [29] , we thus infer that the quasi-amorphous MoS 2 modification may benefit the hybrid material to catalytically evolve H 2 . Energy-dispersive X-ray spectrum (EDX; Fig. 2f ) analysis further confirmed the formation of MoS 2 /CoSe 2 hybrid with Co, Se, Mo and S as the principal elemental components (Cu and C peaks emanate from the carbon-coated TEM grid), agreeing with the X-ray photoelectron spectroscopy (XPS) results ( Supplementary Fig. 7 ). Scanning TEM (STEM) and EDX elemental mappings revealed uniform spatial distribution of Co, Se, Mo and S over the marked detection range of the constructed hybrid material ( Fig. 2g ). Catalytic hydrogen evolution To assess the HER electrocatalytic activity, thin film of various catalysts was prepared on glassy carbon (GC) electrodes for cyclic voltammetry in H 2 -saturated 0.5 M H 2 SO 4 electrolyte (see Methods for experimental details). Potentials were measured vs saturated calomel electrode (SCE) and are reported vs reversible hydrogen electrode (RHE). The electrode was kept rotating (1,600 r.p.m.) during the measurements to remove in situ -emerged H 2 bubbles. 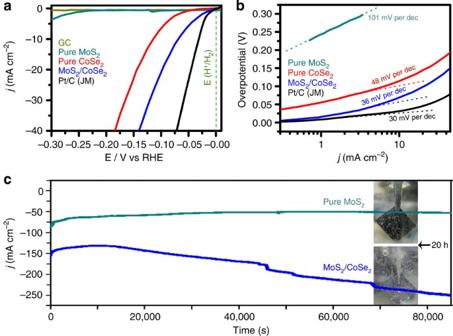Figure 3: Electrocatalytic hydrogen evolution of different catalysts. (a) Polarization curves for HER on bare GC electrode and modified GC electrodes comprising MoS2/CoSe2hybrid, pure MoS2, pure CoSe2and a high-quality commercial Pt/C catalyst. Catalyst loading is about 0.28 mg cm−2for all samples. Sweep rate: 2 mV s−1. (b) Tafel plot for the various catalysts derived froma. (c) Chronoamperometric responses (j~t) recorded on MoS2/CoSe2hybrid and pure MoS2at a constant applied potential of −0.7 V vs SCE. The catalysts were deposited on CFP with the same loading of 1 mg cm−2. Inset digital photos show the H2bubbles formed on MoS2-modified CFP (up) and MoS2/CoSe2-modified CFP (down) at the time point of 20 h. All the measurements were performed in H2-saturated 0.5 M H2SO4electrolyte. dec, decade. Figure 3a shows that GC electrode guarantees a minimal background activity for H 2 evolution. A reductive sweep of MoS 2 /CoSe 2 hybrid showed a low η of 11 mV for the HER, beyond which a sharp increase in cathodic current was observed, corresponding to catalytic H 2 evolution ( Fig. 3a ; Supplementary Fig. 9 ). By contrast, pure CoSe 2 nanobelts exhibited inferior HER activity with a larger onset potential of ~50 mV and lower catalytic current, while pure MoS 2 nanosheet aggregates only affected little HER activity. The HER kinetics of the above catalysts was probed by corresponding Tafel plots (log j ~ η ) ( Fig. 3b ). Tafel slope of ~36 mV per decade was measured for MoS 2 /CoSe 2 hybrid, which is close to the value of 30 mV per decade for Pt/C catalyst and lower than that of 48 mV per decade for CoSe 2 and 101 mV per decade for 3D MoS 2 aggregates ( Table 1 ). This Tafel slope is also comparable to or lower than that of all the reported noble-metal-free HER catalysts in the literature ( Supplementary Table 1 ), demonstrating the superior HER kinetics of MoS 2 /CoSe 2 hybrid. At high current densities (for example, 10 mA cm −2 with η of 68 mV), MoS 2 /CoSe 2 hybrid also represents a more efficient catalyst relative to other noble-metal-free HER catalysts ( Supplementary Table 1 ). The HER inherent activity of these catalysts was evaluated by the exchange current density ( j 0 ). The j 0 of 7.3 × 10 −2 mA cm −2 for MoS 2 /CoSe 2 hybrid outperforms the values of 8.4 × 10 −3 mA cm −2 for pure CoSe 2 and 9.1 × 10 −4 mA cm −2 for pure MoS 2 ( Table 1 ) and also the j 0 value for most of the reported noble-metal-free HER catalysts ( Supplementary Table 1 ). The high electrode kinetic metrics (including onset potential of −11 mV and the Tafel slope of 36 mV per decade) and large j 0 (only ~1 order of magnitude lower than the value of 7.1 × 10 −1 mA cm −2 for Pt) highlight the exceptional H 2 evolving efficiency of the new MoS 2 /CoSe 2 hybrid catalyst. Figure 3: Electrocatalytic hydrogen evolution of different catalysts. ( a ) Polarization curves for HER on bare GC electrode and modified GC electrodes comprising MoS 2 /CoSe 2 hybrid, pure MoS 2 , pure CoSe 2 and a high-quality commercial Pt/C catalyst. Catalyst loading is about 0.28 mg cm −2 for all samples. Sweep rate: 2 mV s −1 . ( b ) Tafel plot for the various catalysts derived from a . ( c ) Chronoamperometric responses ( j ~ t ) recorded on MoS 2 /CoSe 2 hybrid and pure MoS 2 at a constant applied potential of −0.7 V vs SCE. The catalysts were deposited on CFP with the same loading of 1 mg cm −2 . Inset digital photos show the H 2 bubbles formed on MoS 2 -modified CFP (up) and MoS 2 /CoSe 2 -modified CFP (down) at the time point of 20 h. All the measurements were performed in H 2 -saturated 0.5 M H 2 SO 4 electrolyte. dec, decade. Full size image Table 1 Comparison of catalytic parameters of different HER catalysts. Full size table Material stability The long-term stability of MoS 2 /CoSe 2 hybrid catalyst was assayed by means of chronoamperometry measurement ( j ~ t ) with a high catalyst loading of 1 mg cm −2 on carbon fibre paper (CFP). This quasi-electrolysis process was performed at a constant potential of −0.7 V vs SCE in 0.5 M H 2 SO 4 for 24 h. As shown in Fig. 3c , the current density of MoS 2 /CoSe 2 -modified CFP electrode decreased gradually at the initial 3 h, which then increased quickly over 24 h of continuous operation. We hypothesize that the more efficient HER-active sites in our hybrid materials are the interfaces between MoS 2 and CoSe 2 , where Co from the support materials could promote the HER kinetics by lowering the Gibbs free energy of adsorbed hydrogen (Δ G H ) [8] , [29] , [30] . The severe reducing condition at the initial 3 h caused degradation of external MoS 2 and allowed more electrolyte to access the MoS 2 –CoSe 2 interfaces ( Supplementary Fig. 11 ; Supplementary Note 1 ; Supplementary Table 2 ), yielding the increased HER current density. Remarkably, after 24 h of operation, XPS studies revealed no obvious chemical state change of HER-active S ( Fig. 4 ) and the homogeneous elemental distribution was maintained ( Supplementary Fig. 12 ; Supplementary Note 1 ), suggesting the robustness of the hybrid catalyst. By comparison, under the exact same condition, the pure MoS 2 catalyst exhibited a slow but continuous decrease in HER activity. Furthermore, digital photo (inset in Fig. 3c ) taken from MoS 2 /CoSe 2 -modified CFP electrode showed vigorous effervescence at 20 h (also Supplementary Movie 1 ), comparing favourably with the H 2 bubbles formed on free MoS 2 -modified electrode. The exceptional long-term durability of our MoS 2 /CoSe 2 hybrid catalyst suggests the promise for implementing this new catalyst into realistic hydrogen evolution electrode. 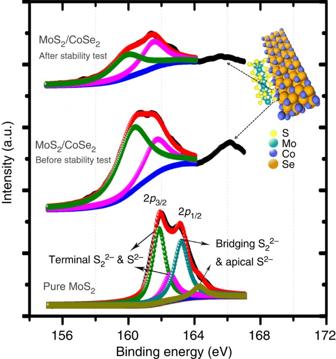Figure 4: S 2pXPS spectrum analysis. S 2pXPS spectra for pure MoS2, MoS2/CoSe2hybrid and MoS2/CoSe2hybrid after stability test. The top right corner demonstrates the structure model of MoS2/CoSe2hybrid. Figure 4: S 2 p XPS spectrum analysis. S 2 p XPS spectra for pure MoS 2 , MoS 2 /CoSe 2 hybrid and MoS 2 /CoSe 2 hybrid after stability test. The top right corner demonstrates the structure model of MoS 2 /CoSe 2 hybrid. Full size image HER-enhanced mechanism The experimentally observed high HER intrinsic activity ( j 0 =7.3 × 10 −2 mA cm −2 ) of MoS 2 /CoSe 2 hybrid catalyst prompted us to probe the enhanced mechanism. Generally, the value of Δ G H is considered as a reasonable descriptor of HER activity for a wide variety of catalysts [3] , [30] , [31] . An optimum HER activity is suggested to be achieved at value of Δ G H ≈0 (ref. 30 ). Lower Δ G H will lead to very high surface coverage of H ads , while higher Δ G H will make the protons bonded too weakly on the catalyst surface, which both lead to the slow HER kinetics [3] , [30] , [31] . Previous density functional theory (DFT) calculations [5] showed that MoS 2 edge sites with unsaturated sulfur atoms can lower the Δ G H approaching to 0 and thus are active for HER, which was later proved by Jaramillo et al. [6] experimentally. Recently, Hu and co-workers [13] , [14] found that amorphous MoS 2 films are particularly HER active and the increased coordinately and structurally unsaturated sulfur atoms led to the enhancement. Furthermore, first-row transition metal ions, especially Co, can promote the HER activity of MoS 2 by coupling with S-edges to lower their Δ G H from 0.18 to 0.10 eV to afford a faster proton adsorption kinetics [8] , [29] , [30] . As to MoS 2 /CoSe 2 hybrid catalyst, the quasi-amorphous MoS 2 around the CoSe 2 may bring in more active edge sites. Meanwhile, the CoSe 2 chemically interacts with MoS 2 by forming S–Co bond ( Fig. 4 and inset), similar to the XPS peak observed in Co-promoted MoS 3 film [32] , which can further improve the HER activity of MoS 2 . By contrast, no such XPS peak was found in Fig. 4 for pure MoS 2 catalyst. XPS analyses of the S 2 p region also exhibit a dramatically decreased electron-binding energy (by ~1.3 eV) after growing MoS 2 on the CoSe 2 , suggesting the formation of more terminal S 2 2− and S 2− ions, which are HER active ( Fig. 4 ) [14] , [19] . Therefore, the CoSe 2 nanobelts, a material with decent HER activity by itself, can not only chemically couple with MoS 2 to promote the HER activity, but also serve as an effective support for mediating the growth of MoS 2 to form more terminal S 2 2− and S 2− . Meanwhile, anchored MoS 2 may also boost the HER-active sites of CoSe 2 and these electrocatalytic synergistic effects [33] together lead to the high HER performance of MoS 2 /CoSe 2 hybrid catalyst. For the HER in acidic media, two separate pathways (the Volmer–Tafel or the Volmer–Heyrovsky mechanism) have been proposed for reducing H + to H 2 (refs 30 , 34 ). Specifically, the two distinct mechanisms involve three principal steps, referring to the Volmer (electrochemical hydrogen adsorption: H 3 O + +e − →H ads +H 2 O), the Heyrovsky (electrochemical desorption: H ads +H 3 O + +e − →H 2 ↑ +H 2 O) and the Tafel (chemical desorption: H ads +H ads →H 2 ↑ ) reactions [30] , [34] . Tafel slope, an intrinsic property of electrocatalysts, could be used to probe the elementary steps involved in the H 2 evolution. For example, HER kinetic models suggest that Tafel slope of about 120, 40 or 30 mV per decade will be obtained if the Volmer, Heyrovsky or Tafel reaction is the rate-determining step, respectively [34] . The Tafel slope down to ~36 mV per decade for MoS 2 /CoSe 2 in 0.5 M H 2 SO 4 is the lowest value measured till now for MoS 2 -based HER catalysts ( Supplementary Table 1 ), even approaching to that of ~30 mV per decade for Pt/C catalysts. This Tafel slope suggests a Tafel-step-determined Volmer–Tafel mechanism works in the MoS 2 /CoSe 2 catalyst, where the synergistic CoSe 2 substrate with decent HER activity presumably contributes to this HER mechanism. Considering that at least one decade of linearity in Tafel extrapolation at relatively large η is desirable to ensure an accurate Tafel analysis, the calculated Tafel slopes ( Fig. 3b ) and derived HER mechanism may be inconclusive. To prove the proposed HER mechanism, we performed a computational study on the new MoS 2 /CoSe 2 catalyst to gain detailed insights into the adsorption, activation and reaction processes ( Fig. 5 ; see Supplementary Methods for computational details). DFT calculations suggested that reactant ( R ) contains two H atoms adsorbed on different sites of the optimized MoS 2 /CoSe 2 model with H–H distance of 2.134 Å. Two approached H atoms on the side S atoms of MoS 2 cluster then formed a transition state ( TS ) with H–H distance of 0.945 Å and imaginary vibration frequency of 828 i cm −1 . After crossing the TS , product ( P ) with a weakly absorbed H 2 molecule (0.745 Å) was formed. The calculated activation barrier of 1.13 eV (30.7 kcal mol −1 ) for the Tafel-step reaction on MoS 2 /CoSe 2 hybrid, which can be overcome at a slightly higher η , approaches that of Pt (111) electrode [35] , agreeing well with our experimentally observed fast HER kinetics. 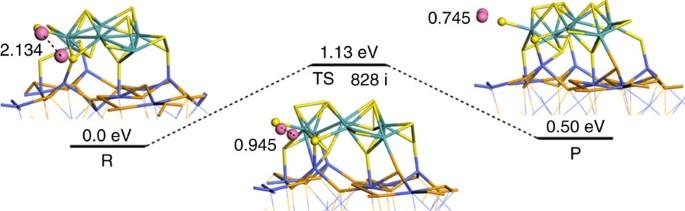Figure 5: HER mechanism. Reaction pathway of HER on MoS2/CoSe2hybrid according to the Volmer–Tafel route. The calculated distance of two hydrogen atoms and energies are displayed in Å and eV. Blue, orange, azure, yellow and pink indicate Co, Se, Mo, S and H atoms, respectively. Figure 5: HER mechanism. Reaction pathway of HER on MoS 2 /CoSe 2 hybrid according to the Volmer–Tafel route. The calculated distance of two hydrogen atoms and energies are displayed in Å and eV. Blue, orange, azure, yellow and pink indicate Co, Se, Mo, S and H atoms, respectively. Full size image In conclusion, we demonstrate that an effective and robust hydrogen evolution catalyst can be made by marrying inexpensive transition metal chalcogenides. The new MoS 2 /CoSe 2 catalyst shows exceptional HER catalytic properties in acidic electrolyte with onset potential of mere −11 mV, a small Tafel slope of 36 mV per decade and a high exchange current density, representing the first non-noble metal catalyst that approaches the performance of state-of-the-art Pt/C catalyst. Inspired by the Nature using transition metals as catalytically active site to construct effective HER catalysts (for example, hydrogenase enzymes) [5] , [36] , we believe that our study here will facilitate the development of newly efficient HER catalysts based on transitional metal chalcogenides. Synthesis of CoSe 2 /DETA nanobelts and MoS 2 /CoSe 2 hybrid All chemicals are of analytical grade and were used as received without further purification. First, ultrathin lamellar mesostructured CoSe 2 /DETA nanobelts were prepared by our recently developed method [20] . Briefly, 0.249 g Co(OAc) 2 ·H 2 O and 0.173 g Na 2 SeO 3 were added into a mixed solution (40 ml) with a volume ratio of V DETA / V DIW =2:1 (DIW, deionized water). The obtained wine solution was then transferred into a 50 ml Taflon-lined autoclave, which was sealed and maintained at 180 °C for 16 h. The resulting black floccules were collected by centrifugation (4,000 r.p.m. for 5 min) and washed by absolute ethanol for three times, and the resulting CoSe 2 /DETA nanobelts were dried for next use. To prepare the MoS 2 /CoSe 2 hybrid, 10 mg freshly made CoSe 2 /DETA nanobelts and 10 mg (NH 4 ) 2 MoS 4 were dispersed in 10 ml DMF and sonicated for 15 min under ambient conditions. Then, 0.05 ml N 2 H 4 ·H 2 O was added into the suspension. After sonicating for another 15 min to dissolve completely, the mixed solution was transferred into a 50 ml Teflon-lined autoclave, which was sealed and heated in an oven at 200 °C for 10 h and then cooled to room temperature naturally. The resulting black product was collected by centrifugation (7,000 r.p.m. for 8 min), then washed at least four times by distilled water and absolute ethanol to remove ions and possible remnants, and dried under vacuum at 80 °C for 6 h. Synthesis of free 3D MoS 2 sheet aggregates The synthetic procedure of free 3D MoS 2 sheet aggregates is the same with that for preparing MoS 2 /CoSe 2 hybrid, the only difference is that no CoSe 2 /DETA nanobelt substrates were added during the synthesis. Characterization The samples were characterized by different analytic techniques. X-ray powder diffraction (XRD) was carried out on a Rigaku D/max-rA X-ray diffractometer with Cu Ka radiation ( λ =1.54178 Å); TEM images, HRTEM images, SAED and an energy-disperse X-ray spectrum (EDS) were taken with a JEOJ-2010 transmission electron microscope with an acceleration voltage of 200 kV. STEM and EDX elemental mapping were performed on JEOL ARM-200F. The X-ray photoelectron spectra (XPS) were recorded on an ESCALab MKII XPS using Mg Ka radiation exciting source. The Fourier transform infrared spectra were measured on a Bruker Vector-22 FT-IR spectrometer at room temperature. Nitrogen sorption was determined by Brunauer, Emmett and Teller measurements with an ASAP-2020 surface area analyzer (see Supplementary Fig. 8 for results). The degradation of external MoS 2 around CoSe 2 was determined by the inductively coupled plasma–atomic emission spectrometry analysis using an Atomscan Advantage (Thermo Ash Jarrell Corporation, USA) spectrometer. Electrocatalytic study Electrochemical measurements were performed at room temperature using a rotating disk working electrode made of GC (PINE, 5 mm diameter, 0.196 cm 2 ) connected to a Multipotentiostat (IM6ex, ZAHNER elektrik, Germany). The GC electrode was polished to a mirror finish (No. 40-6365-006, Gamma Micropolish Alumina, Buehler; No.40-7212, Microcloth, Buehler) and thoroughly cleaned before use. Pt wire and SCE were used as counter and reference electrodes, respectively. The potentials reported in our work were vs the RHE through RHE calibration described below. The preparation method of the working electrodes containing investigated catalysts can be found as follows. In short, 5 mg of catalyst powder was dispersed in 1 ml of 3:1 v/v DIW/isopropanol mixed solvent with 40 μl of Nafion solution (5 wt%, Sigma-Aldrich), then the mixture was ultrasonicated for about 30 min to generate a homogeneous ink. Next, 10 μl of the dispersion was transferred onto the GC disk, leading to the catalyst loading ~0.28 mg cm −2 . Finally, the as-prepared catalyst film was dried at room temperature. For comparison, bare GC electrode that has been polished and cleaned was also dried for electrochemical measurement. Before the electrochemical measurement, the electrolyte (0.5 M H 2 SO 4 ) was degassed by bubbling pure hydrogen for at least 30 min to ensure the H 2 O/H 2 equilibrium at 0 V vs RHE at a rotation rate of 1,600 r.p.m. The polarization curves were obtained by sweeping the potential from −0.7 to −0.2 V vs SCE at room temperature and 1,600 r.p.m. (to remove the in situ -formed H 2 bubbles on the RDE), with a sweep rate of 2 mV s −1 . The electrochemical impedance spectroscopy measurement was performed in the same configuration at open circuit potential over a frequency range from 100 kHz to 5 mHz at the amplitude of the sinusoidal voltage of 5 mV and room temperature (see Supplementary Fig. 10 for results). MoS 2 /CoSe 2 and pure MoS 2 -coated CFPs (Toray, 1 cm 2 , catalyst loading 1 mg) were used as working electrodes to collect chronoamperometry data at the applied potential of −0.7 V vs SCE. The polarization curves were replotted as overpotential ( η ) vs log current (log j ) to get Tafel plots for assessing the HER kinetics of investigated catalysts. By fitting the linear portion of the Tafel plots to the Tafel equation ( η = b log ( j )+ a ), the Tafel slope ( b ) can be obtained. All data were reported without iR compensation. RHE calibration In all measurements, we used SCE as the reference electrode. It was calibrated with respect to RHE. The calibration was performed in the high-purity hydrogen-saturated electrolyte with a Pt foil as the working electrode. Cyclic voltammetry was run at a scan rate of 1 mV s −1 , and the average of the two potentials at which the current crossed 0 was taken to be the thermodynamic potential for the hydrogen electrode reaction. In 0.5 M H 2 SO 4 solution, E RHE = E SCE +0.28 V. DFT calculations The computational modelling of the adsorption, activation and reaction processes involved in HER on MoS 2 /CoSe 2 was performed by periodic DFT with the Vienna Ab-initio Simulation Package (VASP). MoS 2 /CoSe 2 model-building details ( Supplementary Figs 13–15 ), HER mechanism and relevant references are provided in the Supplementary Methods . How to cite this article: Gao, M.-R. et al. An efficient molybdenum disulfide/cobalt diselenide hybrid catalyst for electrochemical hydrogen generation. Nat. Commun. 6:5982 doi: 10.1038/ncomms6982 (2015).